Atroposelective hydroarylation of biaryl phosphines directed by phosphorus centres Prized for their ability to generate chemical complexity rapidly, catalytic carbon–hydrogen (C–H) activation and functionalization reactions have enabled a paradigm shift in the standard logic of synthetic chemistry. Directing group strategies have been used extensively in C–H activation reactions to control regio- and enantioselectivity with transition metal catalysts. However, current methods rely heavily on coordination with nitrogen and/or oxygen atoms in molecules and have therefore been found to exhibit limited generality in asymmetric syntheses. Here, we report enantioselective C–H activation with unsaturated hydrocarbons directed by phosphorus centres to rapidly construct libraries of axially chiral phosphines through dynamic kinetic resolution. High reactivity and enantioselectivity are derived from modular assembly of an iridium catalyst with an endogenous phosphorus atom and an exogenous chiral phosphorus ligand, as confirmed by detailed experimental and computational studies. This reaction mode significantly expands the pool of enantiomerically enriched functional phosphines, some of which have shown excellent efficiency for asymmetric catalysis. Generation of enantiopure molecules that operate efficiently with ideal atom and step economy is a long-standing challenge in organic synthesis [1] , [2] , [3] . Catalytic asymmetric C–H activation [4] , [5] , [6] , [7] , [8] , [9] , [10] , [11] , [12] , [13] , [14] provides a reliable solution to this challenging task. Since a complex molecule typically contains multiple C–H bonds with comparable strengths and steric environments, the most successful method for this transformation is the use of a directing group [15] , [16] , either inherent or preinstalled in organic molecules, to position the metal catalyst at a particular C–H bond in a chiral environment (Fig. 1a ) [17] , [18] , [19] , [20] . In this context, treatment of chiral ligands with metal catalysts has proven to be extremely effective when directed by aromatic nitrogen heterocycles [21] , [22] , carbonyl groups [23] , [24] , [25] , and amino derivatives [26] , [27] . Compared to oxygen and nitrogen atoms, phosphorus coordinates strongly with transition metals and is therefore challenging to use as a director in catalytic C−H activation [28] . Substantial progress has been made in ligand modification through phosphorus-directed C−H activation [29] , [30] , [31] , [32] , [33] , [34] , [35] , [36] , [37] , [38] , [39] , [40] , [41] . We have also demonstrated the viability of using phosphorus directing groups for the site-selective C−H functionalization of indoles at the benzene core [42] , [43] . Despite these advances, asymmetric C−H activation directed by a phosphorus center has not yet been overcome. Fig. 1: Background and discovery. a Pioneering examples of catalytic enantioselective C–H activation assisted by various directing groups. b State-of-the-art methods for catalytic asymmetric synthesis of chiral biaryl phosphines by O-directed C−H activation. c Enantioselective P(III)-directed C−H activation enabled by chiral phosphorus ligands. Full size image Chiral biaryl phosphines are a class of promising ligands and organocatalysts and have become tremendously important in modern organic chemistry [44] , [45] , [46] , [47] . Preparations of these molecules typically require multistep syntheses, in which chiral auxiliaries and kinetic resolution are used most often in practice [48] , [49] . Palladium-catalyzed asymmetric C–C [50] , [51] , [52] and C–P [53] , [54] coupling of aryl (pseudo)halides have been disclosed for the synthesis of axially chiral phosphines. More recently, a series of catalytic asymmetric C–H activation strategies have also been developed to build the biaryl phosphines (Fig. 1b ) [55] , [56] , [57] , [58] , [59] . However, the directing group in these methods is limited to O atom, and additional step for reduction of the formed phosphine oxides is needed. We reasoned that the development of a general strategy to enantioenriched phosphorus ligands through one-step syntheses would likely have a broad impact on asymmetric catalysis. Herein, we report that libraries of chiral biaryl phosphines can be generated by C–H activation with high regio-, stereo- and enantioselectivity (Fig. 1c ). Chirality transfer occurs by combining a metal catalyst with a phosphorus directing group and a chiral phosphorus ligand. The main challenges for this process include strong background reactions with stoichiometric phosphines leading to racemization and formation of a thermodynamically stable metal-ligand complex resulting in low conversion. Therefore, the metal catalyst must distinguish between these two different phosphorus atoms and form a high equilibrium population of the required intermediates to achieve good outcome. Reaction design We started our project by identifying a class of biaryl phosphines for asymmetric C–H activation with unsaturated hydrocarbons, which would enable access to atropisomers through dynamic kinetic resolution [60] , [61] . 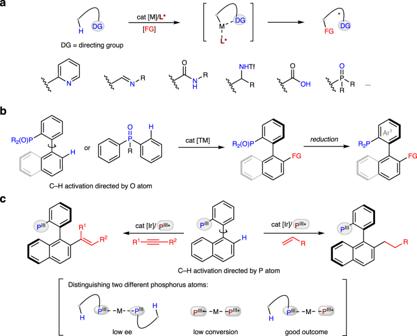Fig. 1: Background and discovery. aPioneering examples of catalytic enantioselective C–H activation assisted by various directing groups.bState-of-the-art methods for catalytic asymmetric synthesis of chiral biaryl phosphines by O-directed C−H activation.cEnantioselective P(III)-directed C−H activation enabled by chiral phosphorus ligands. Phosphine 1a fulfils this criterion and exhibits a barrier of 22.0 kcal/mol for atropisomer interconversion and a sufficiently high rotational barrier for formation of olefination product 3aa (~45 kcal/mol) from alkyne 2a (Table 1 ). When the reaction was conducted with [Ir(cod)Cl] 2 (5.0 mol%) as a catalyst and chiral diene L1 [62] as a ligand in toluene at 70 °C under a N 2 atmosphere, the desired product 3aa was formed in racemic with 33% yield (entry 1). The reaction was then investigated by using the iridium catalyst with a variety of chiral ligands to obtain the enantioselectivity. The use of Carreira ligand L2 led to product 3aa in 79% yield with 51% ee (entry 3). Changing the ligand to the chiral spiro phosphoramidite L3 provided superior results with alkyne 2a , delivering product 3aa in 82% yield and 97% ee (entry 3). Here the absolute stereochemistry of product 3aa was determined by X-ray crystallographic analysis. Loading the BINOL-derived phosphoramidite L3 bearing an NMe 2 motif decreased the enantioselectivity to 66% (entry 4). However, treatment of a TADDOL-derived ligand L5 in the system became very sluggish, leading to product 3aa only in trace amounts (entry 5). Other solvents, such as THF and DCM gave much lower enantioselectivities and yields (entries 6-7). Conducting the reaction at 90 °C further improved the yield of 3aa to 88% yield but with a reduced enantioselectivity (entry 8). Low efficiency was observed by conducting the reaction at room temperature (entry 9). It is noteworthy that other iridium sources like [Ir(coe) 2 Cl] 2 also maintained an acceptable enantioselectivity (entry 10), but other transition metals such as [Rh(cod)Cl] 2 gave a remarkably reduced ee value (entry 11) and Pd(OAc) 2 completely failed (entry 12). Decreasing the [Ir(cod)Cl] 2 loading to 2.5 mol% led to a substantial decrease in the yield (entry 13), and a control experiment revealed that the reaction did not proceed without the metal catalyst (entry 14). Table 1 Optimization of the reaction conditions. a Full size table Scope of the methodology With the optimal reaction conditions in hand, we evaluated the scope of two components in this reaction (Fig. 2 ). The scope of phosphines 1 was first examined with alkyne 2a . Phosphines with electron-donating groups, including methyl ( 1b - e ), phenyl ( 1f ) and ether ( 1g - i ) substituents at the P-phenyl ring or naphthalene ring, all delivered excellent enantioselectivities for both hydroarylation reactions. Electron-withdrawing substituents, such as F ( 1j - k ), Cl ( 1l - m ) and CF 3 ( 1n-o ), also worked well. Given the steric requirements of ligands, we further surveyed reactants with in creasingly bulky backbones. Phosphines bearing 1,2-dihydroacenaphthyl ( 1p ), phenanthrenyl ( 1q ), pyrenyl ( 1r ) and a 1,2’-binaphthalenyl ( 1s) motif did not noticeably affect the reaction efficiency and enantioselectivity for either set of reaction conditions. We were pleased to find that heteroaryl-based phosphines, such as quinolone ( 1t ) and dibenzo[ b , d ]furan ( 1u ) were very well tolerated in enantioselective olefination. The reaction of alkyne 2a with N -aryl pyrrole-based phosphine 1v delivered the desired product 3va in 69% yield and 96% ee, showing the same absolute configuration as the biaryl substrates. In addition, variations in the aryl substituents ( 1w ) at the phosphorus atom with different electronic properties, were well tolerated under reaction conditions. Furthermore, a thiophenl-containing ligand 1x also proved to be highly efficient. We then explored the scope for alkynes 2 with the developed conditions. Increasing the steric hindrance in the internal alkynes ( 2b - d ) with ethyl to isobutyl groups maintained the high enantioselectivities but resulted in a gradual decrease in the reaction yield. Nonsymmetric alkynes, such as prop-1-yn-1-ylbenzene ( 2e ), led to enantioenriched product 3ae in a highly regioselective manner, albeit with diminished yield. In addition, the employment of a terminal alkyne 2f as a substrate completely failed to undergo C–H activation in the current system. Fig. 2: Atroposelective P(III)-directed C–H olefination of biaryl phosphines with alkynes. Reaction conditions: [Ir(cod)Cl] 2 (5 mol%), L3 (11 mol%), 1 (0.2 mmol), 2 (1.0 mmol) in 2 mL of dry toluene at 70 °C for 72 h under argon; ee was determined by chiral HPLC analysis; Isolated yield. a At 75 °C. b At 90 °C. Full size image Hydroarylation of biaryl phosphines with olefins was then studied in the transformation (Fig. 3 ). Initially, the different ligands and reaction parameters were evaluated with phosphine 1a and olefin 4a (Fig. 3a ). We found that the selection of the BINOL-derived phosphoramidite L4 under 150 °C for 48 h could give the desired product 5aa (with ~44.8 kcal/mol rotational barrier) in 77% yield and 91% ee. The absolute configuration of this product was confirmed by X-ray diffraction, and the stereochemistry of other products was assigned by analogy to this crystal. Using the same substrates as in Fig. 2 , we next evaluated the reaction efficiency with alkene 4a (Fig. 3b ). A wide range of biaryl phosphines that incorporate electron-neutral ( 1b - e ), electron-donating ( 1f - i ) and electron-withdrawing ( 1j - o ) substituents, were readily tolerated with alkene 4a to produce the related products 5ba - oa in modest to good yields and with excellent levels of enantioselectivities. Moreover, the use of polycyclic phosphine 1p-s and heterocycle-containing phosphines 1t-u did not interfere with productive atroposelective hydroarylation. However, the pyrrole-based phosphine 1v only delivered the desired product 5va in trace amounts at the current reaction conditions. Phosphines 1w-x with different substituents at the P atom were also compatible with this reaction. In addition to alkene 4a , we found that steric hindrance of the acrylate ( 4b-d ) had a minimal impact on the reaction outcome, but styrene ( 4e ) was not compatible with this C–H activation process. Finally, one example highlights the kinetic resolution of racemic 1,1’-binaphthalenyl phosphine 1y by asymmetric hydroarylation of alkene 4a (Fig. 3c ). Chiral product 5ya was formed in 93% ee, and the remaining starting material 1y exhibited an excellent selectivity factor ( S = 99). Fig. 3: Atroposelective P(III)-directed C–H alkylation of biaryl phosphines with alkenes. a Atroposelective hydroarylation of phosphine 1a with olefin 4a . b Reaction substrate scope. c , Kinetic resolution of racemic phosphine 1y by hydroarylation of olefin 4a . Reaction conditions: [Ir(cod)Cl] 2 (5 mol%), L4 (11 mol%), 1 (0.2 mmol), 4 (1.0 mmol) in 2 mL of dry toluene at 150 °C for 48 h under argon; ee was determined by chiral HPLC analysis; Isolated yield. a Using 10.0 equiv. of 4 . Full size image Synthetic applications To emphasize the practicality of our chemistry, we chose some chiral products, including 3aa, 5aa and 5ya , with different steric and electronic properties, to generate a ligand library and tested them for asymmetric catalysis. In the first example (Fig. 4a ), use of 3aa as a ligand in the rhodium-catalyzed arylation of isatin 6 with boronic acid 7 afforded alcohol 8 with good yield and high ee (91%, 93% ee); these were much higher than those obtained using the original MeO-MOP ligand (72%, 75% ee) [63] . In the second case (Fig. 4b ), compound 5aa showed high reactivity for palladium-catalyzed asymmetric allylic alkylation [64] with substrate 9 and dimethyl malonate ( 10 ), which afforded the desired product 11 in 93% yield and with 92% ee. In the third example (Fig. 4c ), phosphine 5ya was used as a ligand for palladium-catalyzed Suzuki-Miyaura cross-coupling of aryl halide 12 with boronic acid 13 to form atropisomeric biaryl 14 in 80% yield and with 93% ee [50] , [51] . These in situ-modified chiral ligands have proven valuable in accelerating the optimization of asymmetric catalysis. Fig. 4: Applications of the developed chiral phosphines in asymmetric catalysis. a Asymmetric aryl-addition reaction. b Asymmetric allylic alkylation reaction. 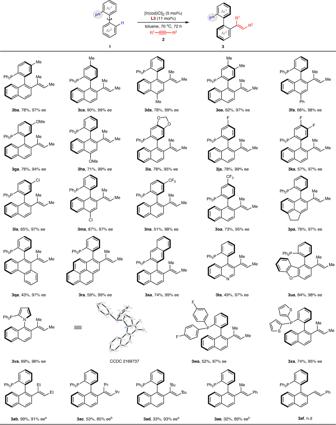Fig. 2: Atroposelective P(III)-directed C–H olefination of biaryl phosphines with alkynes. Reaction conditions: [Ir(cod)Cl]2(5 mol%),L3(11 mol%),1(0.2 mmol),2(1.0 mmol) in 2 mL of dry toluene at 70 °C for 72 h under argon; ee was determined by chiral HPLC analysis; Isolated yield.aAt 75 °C.bAt 90 °C. c Asymmetric Suzuki-Miyaura cross-coupling reaction. Full size image We next performed several experiments to investigate this asymmetric C–H activation. Reacting 1.0 equiv. of L3 with a stoichiometric quantity of [Ir(cod)Cl] 2 yielded complex 15 , as confirmed by X-ray analysis (Fig. 5a ). Using 15 as the catalyst for hydroarylation of alkyne 2a with phosphine 1a yielded compound 3aa with good efficiency, and addition of a catalytic quantity of 3aa to the system as a ligand led to low enantioselectivity (Fig. 5b ). These results showed that the formed products did not serve as ligands. Furthermore, a clear linear effect for the reaction of 1a and 2b indicated that only one chiral ligand could coordinate to the Ir center (see the Supplementary Information for details). A series of deuterium labeling experiments were then performed (Fig. 5c ). The reaction of phosphine d- 1a with alkyne 2a resulted in 47% deuterium incorporation at the olefinic position of product 3aa . Further addition of 10 equiv. of D 2 O to the system dramatically improved the level of deuterium incorporation (85% D), suggesting considerable H/D exchange occurred between the trace water in the solvent and the reaction intermediates. In addition, KIE experiments ( k H / k D = 2.03) indicated that C−H bond cleavage was the rate-determining step in the reaction (Fig. 5d ). [65] Fig. 5: Mechanistic experiments. a Isolation of an iridium complex 15 . b Test of the reactivity of 15 and 3aa for C–H activation of 1a . c Observation of H/D exchange during the reaction of d- 1a with alkyne 2a . d Kinetic isotope effect (KIE) experiments. Full size image The asymmetric C–H activation involves a key intermediate INT1-L3 in which the Ir center coordinates with two phosphorus atoms in the ligand and substrate (Ir/ L3 / 1a = 1/1/1). The high equilibrium population of this species can be illustrated by analysis of the frontier molecular orbitals (Fig. 6 ). The main contribution to the unoccupied molecular orbital (LUMO+2) of the intermediate Ir-monomer came from the Ir 5d orbital, which serves as an electronic acceptor for the phosphorus lone pair. The energy difference between Ir-monomer and the phosphorus-occupied molecular orbital (HOMO-1) of 1a was 1.9 eV less than that of the LUMO+2-HOMO-4 gap between Ir-monomer and the chiral ligand L3 (10.6 eV vs . 12.5 eV), suggesting that strong σ donation makes the electron-rich phosphine 1a more likely to coordinate with Ir-monomer . Then, the η 4 -cod ligand dissociates to provide vacancies around the Ir center ( INT1-L3-pre ) to facilitate the coordination of chiral ligand. The Ir 5d occupied molecular orbital (LUMO) of INT1-L3-pre is thermodynamically favorable to interact with the phosphine 3d unoccupied molecular orbital (HOMO) of L3 than with another phosphine ligand 1a (11.3 eV vs . 13.2 eV). This outcome indicates that the second coordination with L3 mainly occurs via π-back bonding, thus stabilizing the formation of intermediate INT1-L3 . Fig. 6: Analysis of frontier molecular orbitals. HF/6-31G(d)-Lanl2DZ/CPCM. Full size image Based on the aforementioned results, the energy profile for the reaction between phosphine 1a and alkyne 2a is shown in Fig. 7a [66] , [67] , [68] , [69] , [70] . Biaryl atropisomers could easily undergo interconversion and the axial chirality of 1a leads to the formation of two enantiomers INT1-L3-R and INT1-L3-S , where INT1-L3-R was set as the relative zero point of Gibbs free energy. The two enantiomers INT1-L3 undergo C–H activation, generating the iridium complex INT2-L3 through a reversible oxidative addition. Subsequent reductive elimination of H–Cl via transition state TS3-L3 reversibly generates intermediate INT3-L3 , and this process is predominantly a H/D exchange with trace water in the solvent. As a competing pathway, insertion of alkyne 2a into the Ir–H bond of INT2-L3-R leads to INT4-L3-R via TS4-L3-R with a relative free energy barrier of 30.7 kcal·mol −1 , which is comparable in energy to the transition state TS3-L3 , but 2.5 kcal·mol −1 lower than that for the formation of INT4-L3-S (30.7 vs 33.2 kcal·mol −1 , Fig. 7b ). The irreversible alkyne insertion has the highest activation energy in the catalytic cycle and is therefore proposed to be the rate-determining and enantio-determining step, in accordance with the results of KIE experiments. The stereochemical model can be further visualized by steric maps around the Ir catalyst using SambVca 2.1 tool (Fig. 7c ). The geometries of TS4-L3-R and TS4-L3-S are octahedron, where Ir–Cl bond is defined as Z axis and chiral ligand L3 is located in SE quadrant of the steric map. In both transition state TS4-L3 s, C–H bond adjacent to the Ir–C bond towards to the direction of Ir–Cl bond and interacts with nitrogen atom of L3 by weak hydrogen bond, resulting L3 appears vertically more extended in favored transition state TS4-L3-R and horizontally more extended in disfavored TS4-L3-S . The horizontal extension increases the repulsion interaction between methyl group of alkyne and phenyl ring of L3 , resulting the energy barrier of TS4-L3-S is significantly higher than that of TS4-L3-R . The dominant intermediate INT4-L3-R further undergoes reductive elimination through transition state TS5-L3-R with an activation free energy of 13.8 kcal·mol −1 to form the INT5A-L3-R complex. Finally, ligand exchange between INT5A-L3-R and phosphine 1a releases product 3aa and regenerate INT1-L3 to complete the catalytic cycle. Fig. 7: Computational investigations. 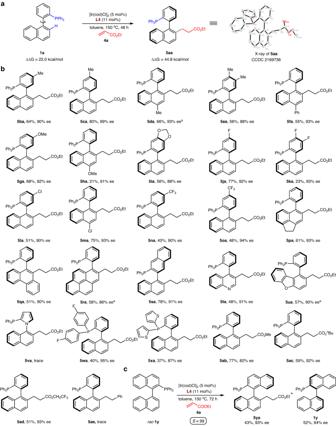Fig. 3: Atroposelective P(III)-directed C–H alkylation of biaryl phosphines with alkenes. aAtroposelective hydroarylation of phosphine1awith olefin4a.bReaction substrate scope.c, Kinetic resolution of racemic phosphine1yby hydroarylation of olefin4a. Reaction conditions: [Ir(cod)Cl]2(5 mol%),L4(11 mol%),1(0.2 mmol),4(1.0 mmol) in 2 mL of dry toluene at 150 °C for 48 h under argon; ee was determined by chiral HPLC analysis; Isolated yield.aUsing 10.0 equiv. of4. a DFT-computed reaction pathways (ωb97xd/6-311+G(d,p)-SDD(Ir)/CPCM//B3LYP-D3BJ/6-31G(d)-Lanl2DZ(Ir)/CPCM). b Stereochemical mode. c Steric maps of the Ir(III) transition states TS4-L3-R and TS4-L3-S . Full size image In summary, we have demonstrated an enantioselective catalytic strategy for phosphorus-directed C–H activation enabled by chiral phosphorus ligands with iridium catalysts. This method represents an effective approach for modular syntheses of chiral phosphorus ligands via one-step transformations with widely available parent ligands, which considerably expands the toolbox of reactions available to synthetic chemists. Furthermore, the results of this study constitute a proof of principle for asymmetric C–H activations in more general molecules, which may furnish solutions for the remaining limitations in this field. 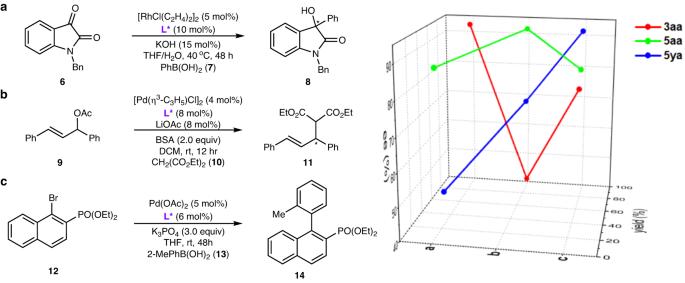Fig. 4: Applications of the developed chiral phosphines in asymmetric catalysis. aAsymmetric aryl-addition reaction.bAsymmetric allylic alkylation reaction.cAsymmetric Suzuki-Miyaura cross-coupling reaction. 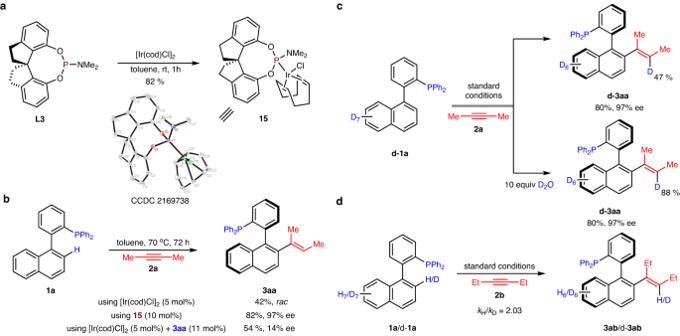Fig. 5: Mechanistic experiments. aIsolation of an iridium complex15.bTest of the reactivity of15and3aafor C–H activation of1a.cObservation of H/D exchange during the reaction of d-1awith alkyne2a.dKinetic isotope effect (KIE) experiments. 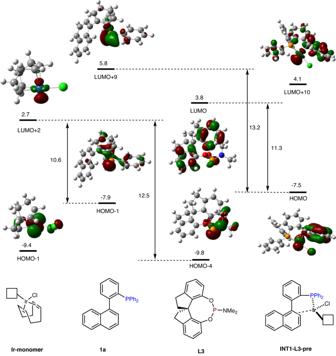Fig. 6: Analysis of frontier molecular orbitals. HF/6-31G(d)-Lanl2DZ/CPCM. 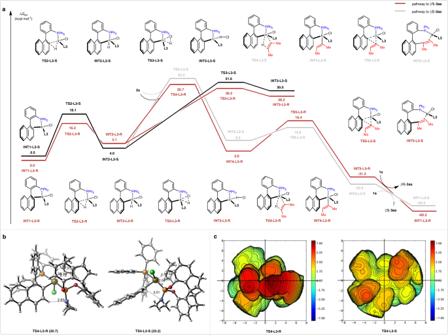Fig. 7: Computational investigations. aDFT-computed reaction pathways (ωb97xd/6-311+G(d,p)-SDD(Ir)/CPCM//B3LYP-D3BJ/6-31G(d)-Lanl2DZ(Ir)/CPCM).bStereochemical mode.cSteric maps of the Ir(III) transition statesTS4-L3-RandTS4-L3-S. Due to slight variations in the experimental protocols for the processes presented herein, we refer the reader to the Supplementary Information for experimental details.